Microbial genomic analysis reveals the essential role of inflammation in bacteria-induced colorectal cancer Enterobacteria, especially Escherichia coli , are abundant in patients with inflammatory bowel disease or colorectal cancer (CRC). However, it is unclear whether cancer is promoted by inflammation-induced expansion of E. coli and/or changes in expression of specific microbial genes. Here we use longitudinal (2, 12 and 20 weeks) 16S rRNA sequencing of luminal microbiota from ex-germ-free mice to show that inflamed Il10 −/− mice maintain a higher abundance of Enterobacteriaceae than healthy wild-type mice. Experiments with mono-colonized Il10 −/− mice reveal that host inflammation is necessary for E. coli cancer-promoting activity. RNA-sequence analysis indicates significant changes in E. coli gene catalogue in Il10 −/− mice, with changes mostly driven by adaptation to the intestinal environment. Expression of specific genes present in the tumour-promoting E. coli pks island are modulated by inflammation/CRC development. Thus, progression of inflammation in Il10 −/− mice supports Enterobacteriaceae and alters a small subset of microbial genes important for tumour development. The microbiota has an essential role in regulating intestinal homeostasis through its capacity to modulate various biological activities ranging from barrier, immunity and metabolic function [1] . Not surprisingly, microbial dysbiosis is associated with numerous intestinal disorders including inflammatory bowel diseases (IBD) and colorectal cancer (CRC) [2] . Whether microbial dysbiosis observed in CRC patients is a consequence of the pathology or is a causal, active modifier of disease outcome remains to be defined. Recent evidence generated from experimental models indicates that microbial dysbiosis can influence intestinal disease, as implantation of cancer-associated biota increased cancer development in the azoxymethane (AOM)/dextran sodium sulphate model of colitis-associated CRC [3] , [4] . At the taxonomic level, analysis of the human CRC microbiome has identified potential microbial candidates implicated in the pathology, including Enterobacteriaceae / E. coli and Fusobacterium [5] . Subsequent experiments using preclinical models of CRC have confirmed the carcinogenetic potential of both Fusobacterium and Enterobacteriaceae / E. coli [6] , [7] , [8] . While the biological events implicated in the development of microbial dysbiosis and emergence of carcinogenic microorganisms are yet to be defined, host genetics and environmental factors such as diet and lifestyle are likely contributing elements in microbial community assembly and maintenance [9] . Chronic inflammation has been recognized as an important risk factor for numerous forms of cancer, including CRC [10] . Importantly, inflammation experienced by IBD patients is associated with a higher abundance of Enterobacteriaceae / E. coli in their intestinal microbiota [11] . In addition, patients with IBD and CRC displayed an increased prevalence of mucosal-associated E. coli compared with non-IBD and non-CRC control subjects [12] , [13] , [14] , [15] . Similarly, in a model of colitis-associated CRC, we have previously observed a higher abundance of Enterobacteriaceae / E. coli in Il10 −/− mice compared with wild-type (WT) controls [6] . While high abundance of Enterobacteriaceae / E. coli appears to be a trademark of IBD, CRC and mouse models of these diseases, it is still unclear if the presence of E. coli at high abundance is sufficient to promote carcinogenesis or whether changes in microbial activities are a necessary step in the pathology. For example, we and others have observed a high abundance of E. coli encoding the genotoxic island pks in the intestine of IBD and CRC patients [6] , [16] , [17] , and found that pks induces double-strand DNA damage in mammalian cells and CRC development in preclinical models [6] , [18] , [19] . Although the presence of pks enhances the cancer-promoting activity of E. coli NC101 (ref. 6 ), the same pks island is necessary for the probiotic (anti-inflammatory) activity of E. coli Nissle 1917 (ref. 20 ). Therefore, it is likely that microbial abundance and gene activities are subjected to complex environmental regulation, which ultimately dictates whether the outcome for the host is beneficial or deleterious. Inflammation has been mostly studied as an environmental factor affecting host physiology and pathology such as cancer development. While recent studies have shown that inflammation fosters the bloom of Enterobacteriaceae [21] , [22] , these studies mostly focused on the behaviour of invading microorganisms in the context of an acute inflammation. In contrast, the interplay between an endogenous microbial community, inflammation and host pathology remains largely undefined. To address this important question, here we longitudinally evaluate microbial community composition in a model of colitis-associated CRC using conventionalized Il10 −/− mice (that is, ex-germ-free mice moved to specific pathogen free housing). In addition, we examine the impact of inflammation on E. coli ’s carcinogenic potential using microbial RNA-sequencing (RNA-seq). Our study indicates that inflammation reduces the strong selection pressure responsible for Enterobacteriaceae / E. coli decline over time. We find that inflammation is essential for E. coli -induced CRC in interleukin 10 ( Il10 )-deficient mice, as the pathology is not observed in inflammation-resistant Il10 −/− ; Rag2 −/− mice. Evaluating the E. coli transcriptome reveals, surprisingly, that E. coli gene expression is most strongly influenced by colonization of the mammalian intestine over time, with only a minimal repertoire of genes influenced by inflammation/cancer, among them the genotoxic island pks . This study demonstrates the dynamic and complex response of commensal microbes to host environmental factors, and illustrates the key role of inflammation in promoting E. coli -associated cancer activity. Microbial assembly changes over time in Il10 − / − versus WT mice We had previously observed alterations to the microbiota of Il10 − / − mice at 20 weeks post conventionalization, a time corresponding to development of colitis-associated CRC [6] . To examine the timeline of microbial changes during development of colitis-associated CRC, we longitudinally collected stools from Il10 − / − and WT mice at 2, 12 and 20 weeks after conventionalization, and performed phylogenic studies. In these experiments, mice were allowed to acquire the microbial community from their cage microenvironment [6] , [23] . To assess the effects of genotype and time on microbial community assembly, we performed principal coordinate analysis (PCoA) using Bray–Curtis dissimilarity at the operational taxonomic unit (OTU) level. We used analysis of similarity, nested on cage to correct for observed cage effects [6] , [23] , to compare overall microbial community composition. At all time points, the microbial community of Il10 − / − colitis-susceptible mice differed significantly from that of healthy WT mice ( Fig. 1a and Supplementary Fig. 1 ). We observed a marked shift in both WT and Il10 − / − microbial communities from 2 to 12 weeks and from 2 to 20 weeks ( Fig. 1a ). The WT community structure appears to stabilize earlier than the Il10 − / − community, as a significant difference is observed in Il10 − / − but not WT animals from 12 to 20 weeks ( Fig. 1a–c ). As inflammation in specific pathogen free (SPF) Il10 −/− mice progresses from an average score of 1 at 2 weeks to a score of 2.25 at 12 weeks and over 3 at 20 weeks [6] , we attribute this differential community structure to the presence of inflammation in Il10 − / − mice. Our mixed linear model (see Methods section and McCafferty et al . [23] ) revealed that time and time × genotype interactions are strongly associated with the structure of the microbial community in our experiment, while genotype displays a smaller but still significant association ( Fig. 1d ). Similarly, differences in microbial richness between the Il10 − / − and WT microbiota became more pronounced over time, with inflammation driving statistically significant differences in the communities at the three time points ( Fig. 1e,f and Supplementary Fig. 1 ). Thus, host genotype (inflammation) and time both appear to influence the assembly of the microbial community. 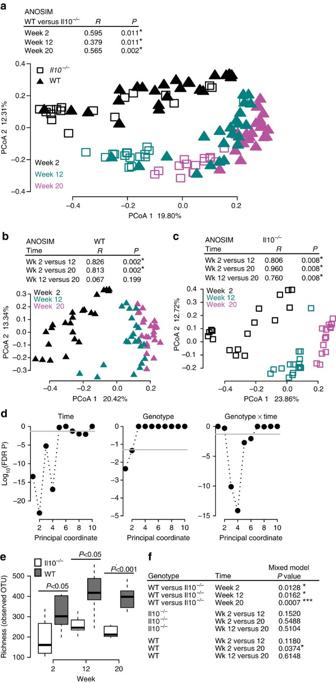Figure 1: Change in microbial community composition over time. (a–c) Bray–Curtis principal coordinate analysis (PCoA) at the operational taxonomic unit (OTU) level, with analysis of similarity (ANOSIM)RandPvalues nested on cage. Each symbol represents an individual mouse at the indicated time point. (d) Mixed linear model FDR-correctedPvalues for the first 10 coordinates of PCoA (explaining 58.4% of the variance), evaluating the null hypothesis that the fixed factor indicated above each plot does not impact the coordinate. Grey line representsP=0.05 significance level. (e,f) Comparisons by the mixed linear model, with all comparisons and FDR-correctedPvalues shown inf.Il10−/−week 2n=17, week 12n=16 and week 20n=15; WT week 2n=24, week 12n=22 and week 20n=24. *P<0.05, ***P<0.001. Figure 1: Change in microbial community composition over time. ( a – c ) Bray–Curtis principal coordinate analysis (PCoA) at the operational taxonomic unit (OTU) level, with analysis of similarity (ANOSIM) R and P values nested on cage. Each symbol represents an individual mouse at the indicated time point. ( d ) Mixed linear model FDR-corrected P values for the first 10 coordinates of PCoA (explaining 58.4% of the variance), evaluating the null hypothesis that the fixed factor indicated above each plot does not impact the coordinate. Grey line represents P =0.05 significance level. ( e , f ) Comparisons by the mixed linear model, with all comparisons and FDR-corrected P values shown in f . Il10 − / − week 2 n =17, week 12 n =16 and week 20 n =15; WT week 2 n =24, week 12 n =22 and week 20 n =24. * P <0.05, *** P <0.001. Full size image Early abundance of Proteobacteria in Il10 − / − mice We and others have observed an increased abundance of Proteobacteria, in particular Enterobacteriaceae and E. coli , associated with IBD and CRC in mice and humans [6] , [12] , [13] , [15] . Therefore, we hypothesized that host-initiated inflammation promotes abundance of Proteobacteria/ Enterobacteriaceae / E. coli , which then supports further inflammation/tumorigenesis. We assessed the phylum level abundance of the luminal microbiota at 2, 12 and 20 weeks post conventionalization. Surprisingly, the abundance of Proteobacteria declined over time as inflammation increases in Il10 − / − mice, although levels are consistently and significantly higher at all time points than in WT mice ( Supplementary Figs 2 and 3 ). A similar phenomenon is observed in WT mice where Proteobacteria declined over time, indicating a natural selection against this phylum over time. In addition, WT mice also exhibited a greater abundance of Bacteroidetes at 2 weeks and a lower abundance of Verrucomicrobia at 12 and 20 weeks, relative to Il10 − / − mice ( Supplementary Fig. 3 and Supplementary Data 1 ). We next assessed the family-level distribution of the microbiota and found that the family Enterobacteriaceae declined over time in both groups, but was significantly more abundant in Il10 − / − relative to WT mice at all time points ( Fig. 2a and Supplementary Data 2 ). At the OTU level, consensus 27, which represents the genera Escherichia/Shigella (99% certainty by Ribosomal Database Project (RDP) classifier), not only displayed a similar pattern of higher abundance in Il10 − / − mice compared with WT but also declined over time ( Fig. 2b ). These data demonstrate similarities in the effect of time on the assembly of the microbiota in both WT and Il10 − / − mice, where there is a shift in community structure over time from an early Firmicutes-dominated community with more Proteobacteria to a community more dominated by Firmicutes and Bacteroidetes with fewer Proteobacteria ( Supplementary Fig. 3 ). Thus, Proteobacteria/Enterobactericeae/ E. coli abundance changes with succession and does not correlate with the progression of inflammation over time. Nonetheless, the abundance of Proteobacteria/ Enterobacteriaceae / E. coli is consistently higher in colitis/cancer-susceptible Il10 − / − mice, relative to WT mice, at all time points ( Fig. 2 ). 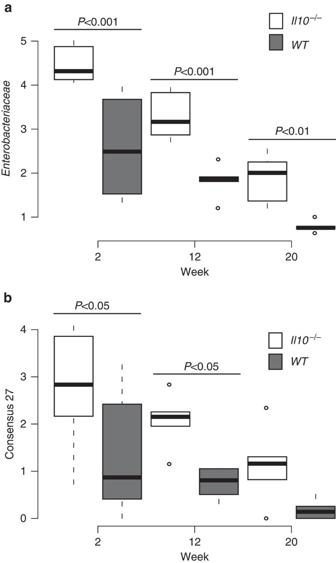Figure 2: Abundance ofEnterobacteriaceaeandEscherichia/Shigella. Increased abundance of (a)Enterobacteriaceaeand (b) OTU consensus 27 (Escherichia/Shigella) inIl10−/−mice. Box and whisker plots show the minimum, first quartile, median, third quartile and maximum relative abundance (showing the median of each cage). FDR-correctedPvalues from the mixed linear model.Il10−/−week 2n=17, week 12n=16 and week 20n=15; WT week 2n=24, week 12n=22 and week 20n=24. Figure 2: Abundance of Enterobacteriaceae and Escherichia/Shigella. Increased abundance of ( a ) Enterobacteriaceae and ( b ) OTU consensus 27 ( Escherichia/Shigella ) in Il10 −/− mice. Box and whisker plots show the minimum, first quartile, median, third quartile and maximum relative abundance (showing the median of each cage). FDR-corrected P values from the mixed linear model. Il10 − / − week 2 n =17, week 12 n =16 and week 20 n =15; WT week 2 n =24, week 12 n =22 and week 20 n =24. Full size image The intestinal E. coli NC101 transcriptome changes over time Having observed that progression of inflammation does not necessarily induce an increase in Enterobacteriaceae abundance, we sought to identify a mechanism by which inflammation is essential for the cancer-promoting activity of E. coli NC101 in AOM/ Il10 − / − mice. We hypothesized that host-initiated intestinal inflammation alters the transcriptional repertoire of E. coli genes that may impact carcinogenesis. We tested this hypothesis by mono-associating germ-free mice with E. coli NC101. In this experimental model, absence of competing microorganisms allows E. coli to maintain a stable niche over time [6] . We then used microbial RNA-seq to evaluate the E. coli transcriptome in stool samples collected over the course of inflammation and tumorigenesis in AOM/ Il10 −/− mice (2 days, and 12 and 18 weeks post mono-association). A principal component analysis (PCA) plot from the normalized counts of all samples and time points revealed a remarkable clustering of the E. coli transcriptome during the progression of inflammation over time ( Fig. 3a ). Numerous genes were differentially expressed (DE) over time (207 from 2 days versus 12 weeks and 1,420 from 2 days versus 18 weeks, false discovery rate (FDR)-corrected P <0.10) and mapping these genes to Kyoto Encyclopedia of Genes and Genomes (KEGG) pathways using Pathview [24] revealed that the majority belong to general metabolic pathways ( Fig. 3b ). From these experimental results, we concluded that these transcriptomic changes over time may be because of the progression of inflammation from 2 days to 18 weeks, or simply represent normal adaptation to the intestinal niche. 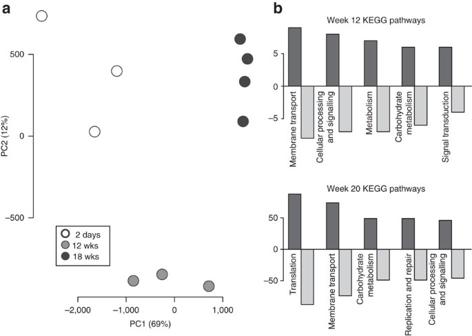Figure 3: RNA-seq reveals changes to theE. colitranscriptome over time in AOM/Il10−/−mice. (a) Principal component analysis (PCA) plot constructed from the normalizedE. coligene counts from AOM/Il10−/−mice at all time points. Each symbol indicates an individual mouse at each time point (white=day 2, grey=week (wk) 12 and black=week 18). (b) Number of DE genes (FDR-correctedPvalue <0.1) in the top five most represented KEGG pathways. Positive values onyaxis represent genes upregulated and negative values represent genes downregulated relative to day 2 time point. Figure 3: RNA-seq reveals changes to the E. coli transcriptome over time in AOM/ Il10 −/− mice. ( a ) Principal component analysis (PCA) plot constructed from the normalized E. coli gene counts from AOM/ Il10 −/− mice at all time points. Each symbol indicates an individual mouse at each time point (white=day 2, grey=week (wk) 12 and black=week 18). ( b ) Number of DE genes (FDR-corrected P value <0.1) in the top five most represented KEGG pathways. Positive values on y axis represent genes upregulated and negative values represent genes downregulated relative to day 2 time point. Full size image E. coli requires inflammation to promote AOM-initiated CRC RNA-seq analysis revealed substantial changes to the E. coli transcriptome over the time of intestinal colonization in Il10 −/− mice ( Fig. 3 ), but it was unclear whether these changes were due to inflammation/cancer or adaptation to the mammalian intestine (that is, colonization time). Moreover, the functional implication for these E. coli transcriptional responses in mediating this carcinogenic effect was unclear. To determine what changes in the E. coli transcriptome are induced by inflammation and may impact the development of CRC, we used Il10 −/− ;Rag2 −/− mice that lack functional T and B cells, which are essential cellular components for development of chronic colitis [25] . One cohort of Il10 − / − mice was not injected with AOM in order to evaluate the pro-carcinogenic effect of E. coli NC101 in the absence of initiation by a carcinogen. Histological analysis revealed high levels of inflammation that did not differ between AOM/ Il10 −/− and Il10 −/− mice, but a complete absence of inflammation in AOM/ Il10 −/− ;Rag2 −/− mice at 20 weeks post colonization ( Fig. 4a ). The number of macroscopic tumours was higher in AOM/ Il10 −/− versus Il10 −/− mice, and invasive tumours (neoplasia score of 4 or 5) were only detected in AOM-treated animals ( Fig. 4b,c ), supporting our earlier observations [6] that E. coli NC101 rarely induces invasive tumours in Il10 −/− mice in the time frame tested. Both AOM/ Il10 −/− and Il10 −/− mice exhibited a significantly higher tumour burden than AOM/ Il10 −/− ;Rag2 −/− mice ( Fig. 4b ). In these nine non-inflamed AOM/ Il10 −/− ;Rag2 −/− mice, four exhibited no macroscopic tumours and five exhibited one non-invasive macroscopic tumour each. In agreement with histological inflammation, expression of inflammatory cytokines was lower in AOM/ Il10 −/− ;Rag2 −/− versus AOM/ Il10 −/− or Il10 −/− mice ( Supplementary Fig. 4 ). Faecal E. coli load did not differ between AOM/ Il10 −/− ;Rag2 −/− , AOM/ Il10 −/− and Il10 −/− mice, as measured by 16S PCR analysis, suggesting that low inflammation and tumour loads in AOM/ Il10 −/− ;Rag2 −/− mice are not due to fluctuation in E. coli NC101 abundance ( Fig. 4d ). These data demonstrate that the sole presence of E. coli is not sufficient to induce CRC in Il10 −/− mice, and that inflammation is essential to the tumorigenic process. 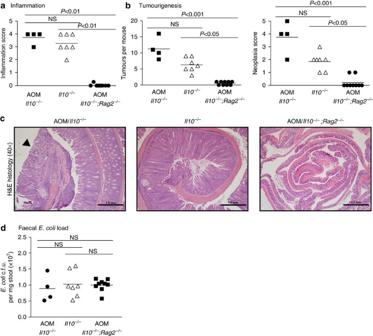Figure 4: Inflammation is required forE. coli-enhanced tumorigenesis inIl10−/−mice. Histologic scoring of (a) inflammation and (b) tumorigenesis. (c) Representative haematoxylin and eosin (H&E) histology at 40 × magnification; scale bars, 1.0 mm; and neoplastic lesion indicated with arrowhead. (d) LuminalE. coliload by qPCR of faecal genomic DNA. (a,b,d) Each symbol represents an individual mouse, line at mean,Pvalues by Kruskal–Wallis with Dunn’s test for multiple comparisons. NS, not significant; c.f.u., colony-forming unit. Figure 4: Inflammation is required for E. coli -enhanced tumorigenesis in Il10 −/− mice. Histologic scoring of ( a ) inflammation and ( b ) tumorigenesis. ( c ) Representative haematoxylin and eosin (H&E) histology at 40 × magnification; scale bars, 1.0 mm; and neoplastic lesion indicated with arrowhead. ( d ) Luminal E. coli load by qPCR of faecal genomic DNA. ( a , b , d ) Each symbol represents an individual mouse, line at mean, P values by Kruskal–Wallis with Dunn’s test for multiple comparisons. NS, not significant; c.f.u., colony-forming unit. Full size image Colonization over time shapes the gut E. coli transcriptome Although we observed substantial changes in the E. coli transcriptome over time in mono-associated AOM/ Il10 −/− mice ( Fig. 3 ), this transcriptional response could be due to either microbial adaptation or inflammation. To control for the effects of time (adaptation), independent of inflammation, we performed microbial RNA-seq analysis on longitudinally collected stool samples from germ-free mice mono-associated with E. coli NC101 with inflammation ( Il10 − / − ), inflammation/CRC (AOM/ Il10 − / − ) and no inflammation/CRC (AOM/ Il10 − / − ; Rag2 −/− ) at 2, 12 and 20 weeks post colonization ( Fig. 5a ). These time points were selected based upon previous observations regarding the development of inflammation (minimal at 2 weeks) and cancer (pre-cancer at 12 weeks and cancer at 20 weeks) in these mice as described above ( Fig. 1 ). To assess the effects of inflammation/genotype and time of colonization on the E. coli transcriptome, we first generated a PCA plot from the normalized gene counts of all the samples and time points. Surprisingly, the E. coli transcriptome clustered predominantly by time of colonization, rather than inflammation/genotype ( Fig. 5b ). This revealed time to be the most significant factor affecting the E. coli transcriptome. We next compared differential gene expression over time between and within each disease group to evaluate E. coli transcriptome changes during adaptation to colonize the mammalian intestine. We found that there were 568–1,000 DE genes within each disease group between 2 and 12 weeks post colonization and 995–1,233 DE genes between 2 and 20 weeks. To determine which changes in gene expression occurred in response to colonization regardless of host genotype/disease, we identified the DE genes common among all three disease groups and found 272 DE genes between 2 and 12 weeks, and 465 DE genes between 2 and 20 weeks ( Supplementary Data 3 ). Mapping these genes to KEGG pathways revealed that the majority belong to general metabolic pathways ( Supplementary Fig. 5 ). These data suggest that E. coli adaptation to the mammalian intestine induces significant changes to the microbial transcriptome. 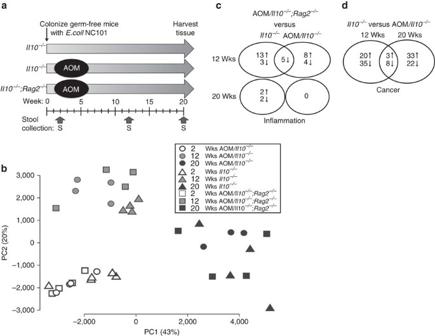Figure 5: Microbial adaptation to the mammalian intestine drivesE. colitranscriptional changes over time. (a) Timeline of sample collection. (b) Principal component analysis plot constructed from the normalizedE. coligene counts from all samples and time points. Each symbol indicates an individual mouse at each time point (white=week (wk) 2, grey=week 12 and black=week 20). Shape indicates genotype/disease: circle=AOM/Il10−/−n=4 (20 weeksn=3), triangle=Il10−/−n=4 and square=AOM/Il10−/−;Rag2−/−n=4. (c,d) Venn diagrams of differential expression (FDR-correctedP<0.10) in (c) AOM/Il10−/−;Rag2−/−versus AOM/Il10−/−orIl10−/−(inflammation), (d) AOM/Il10−/−versusIl10−/−(cancer). Figure 5: Microbial adaptation to the mammalian intestine drives E. coli transcriptional changes over time. ( a ) Timeline of sample collection. ( b ) Principal component analysis plot constructed from the normalized E. coli gene counts from all samples and time points. Each symbol indicates an individual mouse at each time point (white=week (wk) 2, grey=week 12 and black=week 20). Shape indicates genotype/disease: circle=AOM/ Il10 −/− n =4 (20 weeks n =3), triangle= Il10 −/− n =4 and square=AOM/ Il10 −/− ;Rag2 −/− n =4. ( c , d ) Venn diagrams of differential expression (FDR-corrected P <0.10) in ( c ) AOM/ Il10 −/− ;Rag2 −/− versus AOM/ Il10 −/− or Il10 −/− (inflammation), ( d ) AOM/ Il10 −/− versus Il10 −/− (cancer). Full size image The pks genes are DE by cancer status Mono-association experiments indicated that inflammation is necessary for E. coli NC101-enhanced tumorigenesis in AOM-initiated Il10 −/− mice ( Fig. 4 ), which led us to evaluate the effect of inflammation on the E. coli NC101 transcriptome. In this evaluation, we compared gene expression between AOM/ Il10 −/− ;Rag2 −/− (no colitis/baseline reference) versus Il10 −/− (colitis) and versus AOM/ Il10 −/− (colitis/CRC) mice. Surprisingly, few genes were DE in either of these comparisons at any time point ( Fig. 5c and Supplementary Data 4 ). We next evaluated the effect of cancer on the E. coli transcriptome by comparing gene expression between Il10 − / − mice (colitis) versus AOM/ Il10 − / − mice (colitis/CRC). We found that the differential expression of 66 E. coli genes is driven by cancer status at 12 weeks (dysplasia/pre-cancer [6] ) and 20 weeks post colonization (cancer), with 11 of these genes shared among both time points ( Fig. 5d and Supplementary Data 5 ). These differences were unlikely to be caused by AOM treatment alone, as these genes were not DE between Il10 − / − and AOM/ Il10 −/− ;Rag2 −/− mice at 12 or 20 weeks. This suggests that the cancer microenvironment may impact the functional potential of E. coli to promote cancer progression. We have previously shown that disruption of a single gene island, the pks pathogenicity island, can influence the development of cancer in AOM/ Il10 −/− mice [6] . Five pks island genes ( ClbG, ClbH, ClbL, ClbM and ClbN ; Supplementary Data 5 ) were among 66 genes that were significantly impacted by cancer (that is, they were DE between Il10 −/− and AOM/ Il10 −/− ) at 12 weeks ( P <10 − 5 Fisher’s exact test for the null hypothesis that five pks island genes could have been chosen by chance among the 66 DE genes). We used operon-based differential expression analysis (see Methods section) between Il10 −/− and AOM/ Il10 −/− to identify E. coli operons that respond to cancer ( Supplementary Data 6 ). This approach identified the pks island as among the top five operons significantly upregulated (out of 448) in AOM/ Il10 −/− compared with Il10 −/− at 12 weeks time point (FDR-corrected P <0.05). The other four operons identified among the top five DE are ribosomal proteins implicated in housekeeping functions ( Supplementary Data 6 ). Supplementary Figure 6a depicts operons DE on the E. coli NC101 genome and showed the pks island to be one of the most significant responding operons at 12 weeks. At 20 weeks, when cancer has developed, AOM/ Il10 −/− mice show less differential expression of genes in the pks operon (19th most DE, FDR-corrected P =0.73; Supplementary Fig. 6 , right panel). This suggests that changes to the intestinal microenvironment during cancer development may maintain or enhance pks transcription and carcinogenesis/tumorigenesis in carriers of pks + E. coli . Overall, our findings highlight the complex interaction between host inflammation and microbial composition/activity in the development of colitis-associated CRC. We previously reported that intestinal inflammation was not sufficient to promote CRC in Il10 − / − mice, and that specific microbial activities such as those generated by E. coli pks are essential for tumorigenesis [6] . Interestingly, genetic deletion of pks attenuated development of invasive tumours without impacting the colitogenic potential of E. coli , suggesting an uncoupling process between inflammation and carcinogenesis. In this study, we investigated in more detail the relationship between intestinal inflammation and microbial-induced carcinogenic ability. Our work suggests a nuanced relationship between E. coli and inflammation. First, we observed that developing inflammation in Il10 −/− mice is not promoting an expansion of the Enterobacteriaceae / E. coli niche over time, but rather antagonizes the natural negative selection of this bacterial group [23] , [26] , [27] , [28] . This observation is not related to the use of conventionally derived mice, since conventionally raised Tlr5 − / − mice inoculated with E. coli LF82 also exhibited reduced E. coli abundance over time, but still maintained higher levels than non-inflamed mice [29] . Natural negative selection of Proteobacteria is also less efficient in the intestine of human babies with late onset sepsis than in healthy controls [30] . The mechanisms by which E. coli resists negative selection in the inflamed intestinal environment are unclear. A recent report [22] suggested that nitrate production derived from host-inducible nitric oxide synthase (iNOS) fosters the bloom of Enterobacteriaceae . Our observation that there is no correlation between iNOS gene expression and E. coli load, coupled with the protective effect of iNOS in colitis-associated CRC [31] , suggest a more complex interaction between host inflammation, bacteria and tumour development. To determine whether the cancer risk introduced by E. coli is dependent on inflammation, we mono-associated inflammation susceptible AOM/ Il10 − / − and inflammation-resistant AOM/ Il10 − / − ; Rag2 −/− mice with E. coli NC101 and found that a high abundance of E. coli was not sufficient for tumorigenesis in the absence of inflammation. This minimal and non-invasive tumorigenesis is not simply inherent to the Rag2 −/− genotype, as Rag2 −/− mice develop intestinal cancer in response to other stimuli, including the Epsilon-Proteobacteria Helicobacter hepaticus and carcinogen methylcholanthrene [32] , [33] . As E. coli loads were equivalent in inflamed AOM/ Il10 − / − and non-inflamed AOM/ Il10 − / − ; Rag2 −/− mice, the lack of CRC cannot be attributed to a failure to colonize Il10 − / − ; Rag2 −/− mice. Rather, we interpret these findings as meaning that specific environmental conditions (for example, inflammation), in addition to presence of E. coli , are necessary for development of CRC in Il10 − / − mice. We hypothesized that inflammation may alter the gene expression of E. coli during intestinal colonization. However, RNA-seq analysis on longitudinally collected stool samples from inflamed ( Il10 −/− and AOM/ Il10 − / − ) and non-inflamed (AOM/ Il10 − / − ; Rag2 −/− ) mice revealed numerous DE genes and a remarkable clustering of the E. coli transcriptome by time. Thus, microbial adaptation to the mammalian intestine over time—and not mouse genotype and disease phenotype—is a dominant force shaping the intestinal E. coli transcriptome. These results highlight the importance of controlling for the effects of time as well as health and disease phenotypes in order to reach sound conclusions in microbiome studies. Inflammation alters a surprisingly small number of genes at 12 weeks that account for <0.5% of total E. coli genes and virtually no genes (<0.01%) at 20 weeks. It is notable that virtually no gene expression changes are apparent at 20 weeks post colonization, which may indicate that the E. coli transcriptome has adapted to the inflamed intestine after this extended period of colonization. The small number of microbial genes (17–21) regulated by inflammation at 12 weeks sharply contrasts with the 568–1,233 DE genes within each genotype/disease compared across time points. We conclude that at the time points examined in this current study, inflammation minimally impacts E. coli gene expression. Previously, Patwa et al . [34] concluded that inflammation impacts expression of numerous E. coli genes that contrasts with our current findings. This could be owing to profound differences in experimental approach, such as technology (microarray versus RNA-seq), non-inflamed genotype control (WT versus Il10 −/− ;Rag2 −/− ), sampling location (caecal versus faecal) and observation time (single end point versus multiple time points). These mono-association studies may not fully reflect E. coli behaviour in a human host harbouring a naturally acquired complex microbial community. Future studies will determine E. coli transcriptomic response in presence of a complex microbiota. We detected 66 DE genes at both 12 and 20 weeks post colonization in Il10 −/− versus AOM/ Il10 −/− mice, with 11 DE genes represented at both time points throughout the progression of cancer. While it is currently unclear whether these changes are a cause or consequence of cancer development, future functional studies using microbial gene knockouts and gnotobiotic approaches will address the importance of these 11 genes. Indeed our previous work demonstrated that deletion of a single microbial gene cluster, the pks pathogenicity island, can impact the incidence and severity of CRC in E. coli NC101 mono-associated AOM/ Il10 −/− mice [6] . The critical role of pks in promoting CRC was recently confirmed in another experimental model [30] . However, there is no data about the transcriptional regulation of the pks island in vivo during the course of inflammation/cancer. Our data show for the first time that the pks island is significantly responsive to the inflammatory/carcinogenic environment in Il10 −/− mice. Whether other strains harbouring the pks island respond similarly to the inflammatory and carcinogenic environment will require further experiments. At this time, no methods exist to detect the bioactive product of the pks island, colibactin, as its precise structure is unknown, so it is unclear how expression of pks genes relates to the production and cancer-promoting activity of this genotoxin. Nonetheless, maintained expression of genes with cancer-promoting activities could reasonably impact the progression of CRC. In addition to transcriptional response, additional mechanisms could contribute to or modify E. coli carcinogenic potential. For example, many E. coli functions involved in virulence and colonization are a consequence of post-transcriptional regulation (that is, two-component systems [35] , [36] , nucleotide- and small molecule-based second messengers [37] , [38] and so on). Proteomics analysis of E. coli NC101 suggest minimal changes during inflammation [39] . Therefore, it will be important to evaluate the E. coli metabolome in response to inflammation and cancer as metabolomics technologies become better developed and more affordable. Another possible mechanism to be investigated is inflammation-induced loss of protective mucins and increased epithelial access [40] , [41] that can enhance the ability of E. coli to interact with the host epithelium. Defective Muc2 expression in Il10 −/− mice has been shown to facilitate bacterial access to the epithelium [40] , [42] . In this scenario, inflammation would not significantly alter the functional capabilities of E. coli , but would poise it at a unique location with unfettered access to deliver bacterial products to host epithelial cells and impact inflammation and carcinogenesis. This mechanism would be consistent with our observation that non-inflamed AOM/ Il10 −/− ;Rag2 −/− mice fail to develop CRC, despite a high abundance of luminal E. coli. In conclusion, we have found that inflammation does not promote an observable increase in E. coli abundance in the luminal compartment, but may enhance E. coli resilience in the intestine. Although inflammation did not drive substantial changes in the E. coli transcriptome, inflammation was critical for tumour development, perhaps by maintaining expression of selected pks -associated genes. These findings highlight the complex interplay between inflammation, microbial activity and cancer development. Future studies will further elucidate the specific mechanisms by which host and microbial factors produce CRC phenotypes over time. Ethics statement All animal protocols were approved by the Institutional Animal Care and Use Committee of the University of North Carolina at Chapel Hill. AOM/ Il10 − / − model Il10 -deficient, Il10 and recombination activating gene 2 ( Rag2) double-deficient and WT 129/SvEv mice were born and raised in germ-free isolators until either the day they were transferred to SPF facility (SPF model) or mono-associated with E. coli NC101 (mono-association model) for the immediate initiation of CRC experiments. In SPF experiments, mice were colonized by naturally acquiring the microbiota from their cage/room microenvironment upon transfer from germ free (GF) to SPF conditions. This approach negates confounding factors of familial and maternal transmission of the microbiota that can be experienced in mice born and raised in SPF conditions [23] , [43] . Because AOM treatment had no effect on the microbiota assessed at 20 weeks in the previous study [6] ( P =1 using both analysis of similarity and permutational multivariate analysis of variance (PERMANOVA) to evaluate the null hypothesis that AOM does not contribute to microbial community composition in this data set), we did not distinguish between AOM treatment groups in testing hypotheses on the state of the microbial community. For the mono-association model, GF mice were transferred to a gnotobiotic isolator and colonized with E. coli NC101 by gavage and rectal swabbing [44] . They remained in this isolator throughout the study. In all experiments, male and female mice were aged 7–12 weeks at initiation of these experiments and housed 2–4 mice per cage. Four weeks after colonization, mice received 6 weekly intraperitoneal injections of AOM (10 mg kg −1 ). Stool was collected throughout the experiments at 2, 12 and 20 weeks. Mice were killed at 20 weeks, stool and tissue were collected, and colons were examined macroscopically for tumours and then swiss-rolled and fixed in formalin for paraffin embedding and histology [44] . Histology was scored for inflammation [45] and dysplasia/tumours [6] by two blinded experienced investigators. Dysplasia was scored as follows, taking into account the entire colon section and not simply the most severe lesion: 0=no dysplasia, 1=mild dysplasia characterized as aberrant crypt foci, +0.5 for multiples, 2=moderate dysplasia characterized as gastrointestinal neoplasia, +0.5 for multiples, 3=severe or high grade dysplasia characterized as adenoma, restricted to the mucosa, 4=invasive adenocarcinoma, invading into or through the muscularis mucosa, and 5=fully invasive adenocarcinoma, full invasion through the submucosa and into or through the muscularis propria [6] . Animal cohorts Three animal cohorts were used in this manuscript. The first cohort was used for longitudinal sequencing of the faecal microbiota and is described above as the SPF model. 16S data from the 20 weeks time point were previously published [6] . The longitudinal assessment including 2 and 12 weeks time points of this cohort are published for the first time here ( Figs 1 and 2 ). Two additional cohorts, mono-associated with E. coli NC101, were used for RNA-seq and are described for the first time here. One cohort included only AOM/ Il10 −/− mice, with stools from 2 days and 12 and 18 weeks post mono-association used for RNA-seq ( Fig. 3 ). An additional cohort included Il10 −/− , AOM/ Il10 −/− and AOM/ Il10 −/− ;Rag2 −/− mice, with stool samples collected at 2, 12 and 20 weeks post mono-association. In this cohort, cancer and inflammation were assessed ( Fig. 4 ) and RNA-seq was used to evaluate the E. coli transcriptome ( Fig. 5 ). DNA extraction Stool samples were collected from SPF mice to assess luminal microbiota. Colon biopsies (2 × 10 mm) were collected after flushing the colon with phosphate-buffered saline. Samples were immediately stored at −80 °C. DNA was extracted from between 50 and 200 mg of stool or 100 mg colon tissue as described in refs 6 , 44 . Bacterial quantitative quantitative PCR Bacterial quantitative PCR (qPCR) was performed on total DNA extracted from stool at the 20 weeks time point of each experiment as described previously [6] . In brief, amplification was performed in triplicate with SYBR green qPCR chemistry according to the manufacturer’s protocol (Applied Biosystems) using the following primers: E. coli 16S rRNA F 5′- CATGCCGCGTGTATGAAGAA -3′, E. coli 16S rRNA R 5′- CGGGTAACGTCAATGAGCAAA -3′, universal 16S rRNA F 5′- GTGSTGCAYGGYTGTCGTCA -3′, universal 16S rRNA R 5′- ACGTCRTCCMCACCTTCC C -3′ (ref. 6 ). C t values from E. coli were normalized to 16S to generate Δ C t values. E. coli load was calculated by comparing C t values to a standard curve from known concentrations of cultured E. coli NC101. qPCR for host cytokine expression To assess host cytokine expression, RNA was extracted from distal colon biopsies using TRIzol (Invitrogen) and cDNA was reverse transcribed using Moloney murine leukaemia virus (Invitrogen) according to the manufacturer’s instructions. qPCR amplification was performed in triplicate with SYBR green qPCR chemistry (Applied Biosystems) using primers for Nos2 (F-5′- GTGGTGACAAGCACATTTGG -3′, R-5′- GGCTGGACTTTTCACTCTGC -3′) , Il1b (F-5′- GCCCATCCTCTGTGACTCAT -3′, R-5′- AGGCCACAGGTATTTTGTCG -3′) , Ifng( F -5 ′- CTTCCTCATGGCTGTTTCTGG -3′, R-5′- ACGCTTATGTTGTTGCTGATGG -3′), Il12b (5′- GGAAGCACGGCAGCAGCAGAATA -3′ and 5′- AACTTGAGGGAGAAGTAGGAATGG -3′), and Gapdh (F-5′- GGTGAAGGTCGGAGTCAACGGA -3′, R-5′- GAGGGATCTCGCTCCTGGAAGA -3′) on an ABI 7900HT Fast Real-Time PCR System. C t values were normalized to Gapdh to generate Δ C t values, and fold changes were calculated by ΔΔ C t to the mean Δ C t of the AOM/ Il10 −/− ;Rag2 −/− group. Illumina V6 16S library construction and sequencing The V6 hypervariable region of the 16S rRNA gene was amplified using a two-step PCR strategy [6] . The first step uses primers to the V6 region of the 16S rRNA gene that contain a 4–6 nucleotide barcode for multiplexing [6] . The subsequent PCR adds Illumina paired-end sequencing adapters and a flow-cell adapter on the 5′ and 3′ ends of the amplicon. Amplicons were visualized on 1.5% agarose gel and purified using the QIAquick PCR purification kit (Qiagen). A quantity of 50 ng of DNA from each sample was pooled to a final concentration of 29 ng μl and subjected to paired-end Illumina HiSeq2000 sequencing at the University of North Carolina High Throughput Sequencing Facility. A total of 230,348,938 paired-end reads were generated using two lanes of Illumina HISeq2000 for a total of 244 samples. Requiring a minimum of 70 continuous matching nucleotides between the forward and the reverse reads, we generated 40,400,733 consensus sequences for the current study representing 118 samples. Those sequences were processed as described previously [6] , [23] . Abundant OTU+ v.0.93b ( http://omics.informatics.indiana.edu/AbundantOTU/otu+.php ) with the ‘-abundantonly’ option was used to cluster those sequences into 2,273 OTUs incorporating 99.68% of the total input sequences. UCHIME ( http://www.drive5.com/uchime/ [46] ) and the Gold reference database were used to screen for the presence of chimeras in our OTU sequences, and a total of 20 OTUs were removed. The remaining 2,253 OTUs (representing 99.63% of the input sequences) were used for downstream analysis. Taxonomic assignments were done using BLASTn (v. 2.2.28+; ref. 47 ) with an expectation value threshold of e-5 to map the OTU sequences to the Silva database (release 108, http://www.arb-silva.de/ ). After that, we used the standalone version of the RDP classifier (v.2.5; ref. 48 ) to classify the full-length Silva sequences with the best BLASTn match to the OTU sequence requiring an RDP confidence score of ⩾ 80%. Microbial richness was calculated as the number of distinct OTUs present in each sample or each cage (median of all samples from a particular cage) after rarefying to 15,859 sequences/sample or 56,202 sequences/cage. Pivot tables for the OTU, Phylum, Class, Order, Family and Genus were generated as described previously [23] . We used a mixed linear model using SAS software to analyse the data and accounting for possible contributions that may arise from co-housing the mice in the same cage [23] . In Figs 1e and 2 , the median value of each cage is shown for visualization purposes. In Figs 1f and 2 , however, P values are reported from our mixed linear model using F -test, which accounts for the contribution of cage. A parallel analysis using QIIME v.1.7.0 (ref. 49 ) was also conducted, using both de novo (at 97% similarity level) and close-reference OTU picking approaches (at 97% similarity level using the Greengenes 97% reference data set, release of May 2013). This analysis yielded broadly similar results ( Supplementary Fig. 1 ). Bacteria RNA isolation Stool samples were longitudinally collected from Il10 −/− mice at 2 days and 12 and 18 weeks ( Fig. 3 ) or from Il10 −/− , AOM/ Il10 −/− and AOM/ Il10 −/− ;Rag2 −/− mice at 2, 12 and 20 weeks post mono-colonization ( Fig. 5 and Supplementary Fig. 6 ) to isolate bacterial mRNA. Stool samples were snap frozen and stored at −80 °C. RNA was extracted from between 50 and 200 mg of stool as follows. Total bacterial RNA was isolated from stool using RiboPure Bacteria Kit (Ambion, Austin, TX) and depleted of ribosomal and transfer RNA using MicrobeExpress (Ambion). Before preparation of double-stranded cDNA (see below), bacterial DNA contamination was assessed by performing a 50-cycle PCR using 100 ng of RNA as a template with the following primers to detect pks island genes [6] , [50] : clbB forward 5′- GCGCATCCTCAAGAGTAAATA -3′ and reverse 5′- GCGCTCTATGCTCATCAAC -3′ (PCR-product size=283 bp) and clbN forward 5′- GCAGCGCAAAATACCATAAAT -3′ and reverse 5′- TGGGCTGTTGGATTTAGTCAC -3′ (PCR-product size=331 bp). Absence of both bands was required to proceed with the preparation of the double-stranded cDNA. A cDNA library was constructed using TruSeq RNA Sample Prep Kit v2 (Illumina, Hayward, CA). A PCR for clbB and clbN expression was performed (30 cycles) to confirm the presence of these genes on our samples. For the first RNA-seq experiment ( Fig. 3 ), 10 samples were multiplexed into one lane and for the second RNA-seq experiment ( Fig. 5 ), 35 samples were spread into three lanes for paired-end sequencing. One sample from the second RNA-seq experiment could not be assigned to any mouse and therefore was excluded from the analysis. Illumina RNA-seq Our first RNA-seq experiment (AOM/ Il10 −/− ; Fig. 3 ) generated 151,331,485 paired-end reads of 100 bases long for a total of 10 samples. The second RNA-seq experiment ( Fig. 5 and Supplementary Fig. 6 ) generated a total 542,090,141 paired-end reads of 100 bases long for a total of 35 samples. Principal component analysis (PCA) plots revealed no batch effect by lane ( Supplementary Fig. 7 ). A quality control/quality assurance (QC/QA) approach similar to that described by Castellarin et al . [51] was adopted from human to mouse-associated samples to clean and filter the reads. In brief, all reads were mapped to the UCSC mouse genome (mm19) sequences using Novoalign v.2.08.03 (NovoCraft Technologies, Selangor, Malaysia). Reads that mapped to the mouse genome were excluded from further analysis. A re-analysis of the data based on Bowtie2 (ref. 52 ) v. 2.2.1 alignments led to nearly identical results. We screened RNA-seq data for the presence of bacteria other than Escherichia using MetaPhlAn (ref. 53 ) v. 1.7.3, and found that 100% of the reads were assigned to Escherichia except for 3 of 35 samples showing 84%, 93% and 97% of reads assigned to Escherichia . These minority reads were assigned to species that are common contaminants on sequencing equipment: 16% ( Staphylococcus ), 7% ( Staphylococcus ) and 3% ( Pseudomonas ). These data confirm that Il10 −/− mice were only colonized with E. coli . To enhance the available draft genome of E. coli NC101 (NCBI GenBank accession AEFA00000000.1 ), we used reads from the first RNA-seq experiment along with the original Roche 454 sequences that were used to produce the AEFA00000000.1 assembly. The concept of enhancing genome assembly using RNA-seq data has been successfully applied to Caenorhabditis [54] . The RNA-seq reads, from the first RNA-seq experiment, that were used in the genome assembly process were first cleansed (see above) and filtered at Q20, followed by merging overlapping reads using FLASH [55] . Both the merged and unmerged reads were subjected to digital normalization [56] and then fed into Newbler genome assembler (v.2.6 20110517_1502 (ref. 57 )) along with the Roche 454 shotgun sequences. The hybrid assembly reduced the total number of scaffolds from 27 to 10 and increased the N50 value from 511,891 to 848,093 bases. The hybrid assembly was then annotated using Prokka (ref. 58 ) v.1.2. Filtered and cleansed RNA-seq reads were then aligned to this updated draft genome using Novoalign (reference indexed at k-mer length of 10 and step size of 1 using novoindex), resulting in average genome coverage of 16X. Rapaport et al . [59] and Liu et al . [60] have recently shown that the accuracy of gene expression analysis algorithms is enhanced by the number of replicates used (two or three replicates) rather than the coverage depth. Our RNA-seq experiment uses 3–4 replicates; therefore, the accuracy of our differential gene expressions calls should be unaffected by the moderate (16X) coverage depth. Furthermore, MA plots (log 2 fold change versus log 2 mean normalized counts for each transcripts) show that there is no bias in our differential gene expression calls towards the high abundance transcripts ( Supplementary Fig. 8 ). All alignments were sorted by name, indexed and stored in BAM format files. Gene count matrices were generated using htseq-count v.0.5.4p1 ( http://www-huber.embl.de/users/anders/HTSeq/doc/overview.html ) along with the gene transfer format (GTF) file generated from the annotation step above. Differential gene expression was evaluated using edgeR (v.3.2.4; ref. 61 ) according to procedures described in the package’s user guide section 3.3 ( http://www.bioconductor.org/packages/2.12/bioc/html/edgeR.html ). In brief, a contrast matrix incorporating either the time points (for the first RNA-seq experiment) or the genotype/disease groups and the time points (for the second RNA-seq experiment) was generated for each of the comparisons: AOM/ Il10 −/− week 12 versus day 2, AOM/ Il10 −/− week 20 versus day 2 and AOM/ Il10 −/− week 12 versus week 20 (first RNA-seq experiment) or AOM/ Il10 −/− versus Il10 −/− , AOM/ Il10 −/− versus AOM Il10 −/− ;Rag2 −/− and Il10 −/− versus AOM Il10 −/− ;Rag2 −/− (second RNA-seq experiment). Then this contrast matrix was used in gene-wise negative binomial generalized linear model to test the null hypothesis that the contrast (as defined in the contrast matrix) of the coefficients is equal to zero. A gene was considered DE if its FDR-corrected P value was <0.1. Genes were mapped to KEGG pathways using Pathview v. 1.1.7 (ref. 24 ). We performed operon prediction on the filtered and cleansed RNA-seq reads from the second RNA-seq experiment using Rockhopper v.1.2.1 (ref. 62 ); Rockhopper was used for the purpose of operon detection only. We used predicted operons with three or more genes and discarded the rest. Those predicted operons were then used for testing operon differential expression using GAGE v.2.12.0 (ref. 63 ) along with the fitted counts from the binomial generalized linear model of edgeR. All our differential expression analysis was done using edgeR (gene level) or GAGE (operon level). To ensure that the operon prediction algorithm did not unduly influence our results, we repeated our generation of operon P values using a different assembly ( E. coli 536, NCBI GenBank accession NC_008253 ) and its predicted operons from the DOOR2 (ref. 64 ) database. We saw broadly similar results with little pks differential expression at week 2, pks being one of the most upregulated operons at week 12, and a decline in differential expression of pks at week 20 ( Supplementary Fig. 6 ). In determining P values for Supplementary Fig. 6 , only the three animals for which we had RNA-seq data for all three time points were used. We conclude that our results involving pks are not dependent on a particular assembly or operon prediction pipeline. Analysis of the pks pathogenicity island The pks island is composed of ~20 open reading frames spanning ~54 kb (refs 18 , 65 ). It has been shown that the pks island of E. coli strain Nissle 1917 is organized into four polycistronic units: clb C to clb G, clb I to clb N, clb O to clb P and clb R to clb A based on reverse transcription PCR analysis [50] . In our de novo operon prediction, the pks island was organized into two polycistronic units: clb C to clb Q plus two open reading frames predicted as hypothetical proteins and clb R to clb A. When testing for operon differential expression (see above), we ran three analyses; the first using the four polycistronic units from Homburg et al . [50] , the second using the two polycistronic units from Rockhopper predictions and the third using the pks of E. coli 536 as predicted by the DOOR2 database. Statistics Statistical tests are described in figure legends and were computed using PRIMER v. 6, Microsoft Excel, GraphPad Prism, R v.3.0.1 and v.3.0.2 ( http://www.R-project.org ), and/or SAS v. 9.2 and v.9.3 (SAS Institute Inc., Cary, NC). Inflammation, tumorigenesis scoring and qPCR results ( Fig. 4 ) were compared between groups using Kruskal–Wallis with Dunn’s test for multiple comparisons. These tests are two-tailed, α =0.05. We controlled for FDR by correcting the P values using Benjamini and Hochberg [66] approach where applicable. Our mixed linear model, in which genotype and time are fixed effects and cage is a random effect [23] , takes the form of: where Y ijkl represents either PCoA axis value, phylum count, family count, genus count, OTU count or richness value for genotype i , time j , cage k and replicate l . G i is the effect of the i th genotype, were genotype is set to either WT or Il10 −/− . T j is effect from the j th time point. ( GT ) ij is the interaction effect between genotype i and time j . C k(i) is the effect from the k th cage that is nested within the i th genotype and ε ijkl denotes the error associated with measuring Y ijkl . How to cite this article: Arthur, J. C. et al . Microbial genomic analysis reveals the essential role of inflammation in bacteria-induced colorectal cancer. Nat. Commun. 5:4724 doi: 10.1038/ncomms5724 (2014). Accession codes: 16S RNA sequences have been deposited in the MG-RAST database under accession codes 4543412 to 4543529. RNA-seq data have been deposited in the MG-RAST database under accession codes 4544642 to 4544661.